Reply to: Antibiotics and hexagonal order in the bacterial outer membrane 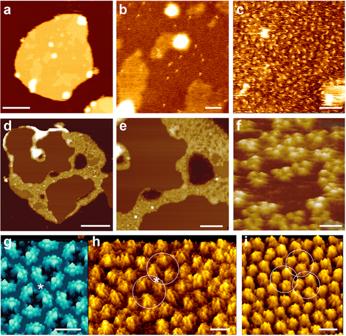Fig. 1: Outer membrane protein assemblies imaged by high-resolution atomic force microscopy (AFM). a–cAFM height images of OMVs collected fromE. colioverexpressing OMPs.aOverview AFM height image of an OMV enriched in the OMP Tsx8. Upon adsorption to mica, the OMVs opened as single layered membrane patches.bRegion from (a) imaged at higher resolution. The membrane contains densely distributed particles protruding from the membrane.cHigh-resolution height image revealing OMPs (single protrusions) in densely packed arrangements.d,eOverview AFM height image of an OMV enriched in the OMP BamA9. The densely packed areas of BamA appear higher (yellow, heights of 10–15 nm) than the surrounding membrane (heights of 5–8 nm).fExtracellular surface of OmpF trimers in a membrane containing lipopolysaccharide (LPS) andE. colilipids7.gExtracellular surface of the atomic model of OmpF trimers rendered at 3 Å (h,i) High-resolution AFM height images of 2D porin OmpF lattices assembled in lipid membranes containing LPS and phospholipids5. The extracellular domains formed by the long OmpF loops protrude by 1.3 nm from the membrane. Shown are OmpF trimers assembled in rectangular (h, 13.5 nm × 8.2 nm) or trigonal (i, 8.2 nm) packing arrangements. AFM images represent height images taken in buffer solution. The brightness range of the AFM height images corresponds to a vertical range of 16 nm (a), 4 nm (b), 1 nm (c), 30 nm (d,e), ≈ 1-2 nm (f) and 1.5 nm (h,i). Height images (f,h,i) are displayed as perspective views. Scale bars, 200 nm (a), 50 nm (b) and 20 nm (c), 160 nm (d), 130 nm (e), 10 nm (f) and 5 nm (g–i). Images were taken from (a–c) ref.8, (d,e) ref.9, (f) ref.7, and (g–i) ref.5. 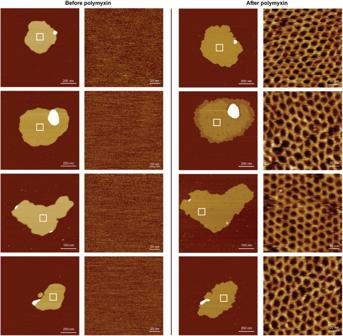Fig. 2: The addition of polymyxin to OMV membranes induces hexagonal assemblies. AFM height images of multiple membranes of OMVs recorded in buffer solution at room temperature. Each OMV membrane is shown before and after the addition of polymyxin. White boxes indicate where AFM height images were recorded to show the appearance of the membrane surface at higher resolution. The absence of structural details indicates that the membrane regions were either devoid of OMPs and contained mainly lipids or that OMPs could not be resolved. Indicative of adding polymyxin to OMV membranes is that they reduce thickness, increase surface area and are covered entirely with hexagonal lattices. OMVs fromE. coliMG1655 WT strain, the AFM sample preparation, and the AFM imaging were prepared as described1. The brightness range of the AFM height images corresponds to a vertical range of 18 nm (overviews) and 2 nm (zoom ins). Scale bars, 200 nm (overviews) and 20 nm (zoom ins). AFM imaging and analysis OMVs produced from different E. coli MG1655 strains were adsorbed onto freshly cleaved mica for 15 min in DPBS buffer at room temperature. After adsorption, the sample was gently washed with fresh DPBS buffer for five times to remove non-adsorbed OMVs. Then OMVs were imaged using force-distance curve-based AFM (FD-based AFM) performed with an AFM (Nanoscope Multimode 8, Bruker) operated in PeakForce Tapping mode in buffer solution (DPBS) at room temperature. The AFM was equipped with a 120 μm piezoelectric scanner and fluid cell. The images were recorded using two different AFM cantilevers: PEAKFORCE‐HiRs‐F‐A (Bruker) with a nominal spring constant of 0.4 N/m, a resonance frequency of ≈165 kHz in liquid, and a sharpened silicon tip with a nominal radius of ≈1 nm or SCANASYST-FLUID + (Bruker) with a nominal spring constant of 0.7 N/m, a resonance frequency of ≈150 kHz in liquid, and a sharpened silicon tip with a nominal radius of ≈2 nm. Before imaging, cantilevers were calibrated by ramping on the mica surface and the thermal tuning method. Images were recorded at 2 kHz oscillation frequency, by applying an imaging force of 100–120 pN with a vertical amplitude of 30 nm. The AFM was placed inside a home‐built acoustic isolated and temperature‐controlled box. Images were collected on a timescale of minutes. Raw AFM images were processed using the AFM analysis software Nanoscope v.1.8 for levelling and flattening.